Synthetic regimes due to packing constraints in dendritic molecules confirmed by labelling experiments Classical theory predicts that branching defects are unavoidable in large dendritic molecules when steric congestion is important. Here we report first experimental evidence of this effect via labelling measurements of an extended homologous series of generations g =1…6 of dendronized polymers. This system exhibits a single type of defect interrogated specifically by the Sanger reagent thus permitting to identify the predicted upturn in the number of branching defects when g approaches g max and the polymer density approaches close packing. The average number of junctions and defects for each member of the series is recursively obtained from the measured molar concentrations of bound labels and the mass concentrations of the dendritic molecules. The number of defects increases at g =5 and becomes significant at g =6 for dendronized polymers where the g max was estimated to occur at 6.1 ≤ g max ≤ 7.1. The combination of labelling measurements with the novel theoretical analysis affords a method for characterizing high g dendritic systems. Intense research efforts are devoted to dendritic molecules comprising of repeatedly branched chains known as dendrons. The dendrons can be attached to point-like cores, to linear polymer chains or to surfaces thus giving rise to three leading structural families of dendritic molecules: dendrimers [1] , [2] , [3] , [4] , [5] , dendronized polymers (DP) [6] , [7] , [8] , [9] and forests [10] , [11] , [12] . Their masses and spans depend on their generation g specifying the number of branching sites along a path between the attachment site and the terminus. The synthesis of ideal dendritic molecules with perfectly regular branching is conceivable for low g values. However, packing constraints rule out such perfect structures at high g when branching defects are unavoidable. The crossover between the two regimes occurs at a theoretically well-defined g max [10] , [12] , [13] , [14] , [15] discussed below. Since the first reports of well-characterized dendrimers in 1985 (refs 16 , 17 , 18 , 19 ), thousands of research articles addressed their synthesis, properties and applications [1] , [2] , [3] , [4] , [5] , [6] , [7] , [8] , [9] , [20] , [21] , [22] , [23] . Recent activity in this area reflects a growing interest in biomedical applications such as bio-imaging, gene and drug delivery [24] , [25] , [26] , [27] , [28] . The overwhelming majority of the literature concerns the g << g max range and highlights structural perfection. In marked distinction, this work focuses on the vicinity of g max , the associated onset of structural imperfection and its characterization. It reports first direct evidence for g max and the associated branching defects. It is enabled by synthesis of a homologous series of DP approaching the vicinity of g max , their characterization and a theoretical framework for quantifying the number of defects. g max of a DP occurs at relatively low values thus rendering the synthesis feasible. The near g max range merits attention for two reasons. First, the existence of the two synthetic regimes is a qualitative signature of dendritic systems that remained essentially unverified and thus of fundamental interest. Second, the exploration of dendritic molecules with g ≥ g max is of practical interest for producing densely packed molecular objects with controllable surface properties and an increased range of tunable spans. Note that while the enhanced tuning range is attained at the price of introducing unavoidable defects at g ≥ g max , there is little evidence that structural perfection is of practical importance. Apart from the pioneering exploration of the near g max range, this work presents a theoretical framework for quantifying defect statistics on the basis of labelling reactions. It thus introduces a simple technique for the detailed quantitative characterization of dendritic molecules. This technique is especially useful at high g and high molecular masses (MM) where the traditional analytical methods are challenged. It is particularly suitable for the study of g max effects diagnosed via defect quantification at high g . The synthetic regimes outlined above reflect a distinctive form of steric hindrance. The term steric hindrance typically connotes the prevention of a chemical reaction by a bulky chemical substituent within a molecule [29] . This local effect assumes a novel, global form in dendritic molecules whereby the overall density within the molecule reduces the reactivity of certain groups [13] . This effect arises in the vicinity of the so-called de Gennes dense packing limit [30] , at , because the bulkier reaction products cannot be accommodated within the available free volume. In turn, the onset of this effect at g max occurs because the mass of an ideal dendron grows exponentially with g while its maximum span increases only linearly [10] , [12] , [13] , [14] , [15] . For g > g max the exponential growth of mass, associated with perfectly regular branching, is impossible. Further growth can only be accommodated by imperfect branching structures leading to sterically induced stoichiometry (SIS) [30] , as was first noted by de Gennes and Hervet in 1983 (ref. 13 ). Since then, the vicinity of g max and the SIS were invoked to rationalize deviations of observed MM from their ideal values [31] , [32] , as well as synthesis failures [33] , [34] , [35] . It was also discussed as a design guideline for controlling the accessibility of the dendritic interior to guest molecules [36] , [37] . With these exceptions, the accumulated evidence of g max and associated SIS since their prediction in 1983 is scanty and indirect. This state is due to a number of difficulties. On the experimental side, studies confront two problems. First, it is synthetically difficult to approach g max for the often studied dendrimers where estimates suggest g max ≈ 10 (refs 13 , 38 ). Second, the observation of g max effects requires quantification of the frequency of branching defects as a function of g over a wide range of g including the vicinity of g max . This is experimentally challenging because the performance of standard characterization techniques, such as nuclear magnetic resonance (NMR) [39] , [40] , [41] , mass spectrometry (MS) [39] and gel permeation chromatography (GPC) [42] , [43] , attain their limits at high g and high MM. While scattering techniques provide information about the dimensions of the dendritic molecules and their density profiles they are not sensitive to branching defects [44] , [45] . On the theory side, computer simulations probed the onset of dense packing in perfect dendritic molecules by monitoring properties such as bond strain and equilibration rates [38] , [46] , [47] . However, these studies do not yield direct information on the occurrence and frequency of structural defects because of their focus on ideally branched structures. In the following, we report a first direct experimental evidence for the existence of two synthetic regimes due to g max effects and SIS in DP. In particular, we focus on the onset of SIS. Attaining this end required two new inputs: a homologous series of DP with an upper g close to g max , and a theoretical method of analysing the defect labelling data to quantify the defect statistics. The two new inputs The first input was enabled by the divergent synthesis of g =6 DP thus producing an extended homologous series of DP with g =1...6, denoted as PG g (Methods). We investigated two homologous series differing in the polymerization degree of the backbone, N : long DP of N≈ 1,000 ( 1,000 PG g ) and short DP with N≈ 45 ( 45 PG g ). The 1,000 PG1... 1,000 PG5 series was reported already [48] , while the 1,000 PG6 and the 45 PG1... 45 PG6 series are new (Methods). As we shall discuss, the differences between the two have a key role in identifying the g max effects and the onset of SIS. The second, theoretical input is the result of an analysis yielding a recursive equation specifying the average number of junctions and termini from measured quantities. With these two inputs at hand, the exploration of g max effects in this system is facilitated by three features (a) g max in long DP occurs at lower g range as compared with dendrimers [10] , [49] . Current estimates for the particular DP studied suggest 6.1 g max 7.1 (ref. 50 ) and thus at the boundary of the g =1...6 homologous series. (b) The DP as synthesized exhibits a single type of defect with no side reactions. In particular, the defect is associated with the occurrence of non-reacted primary amine groups. (c) The number of defects can be quantified via the ultraviolet (UV) absorbance or fluorescence of a label specifically binding to these defects. In this study, the label used is the Sanger reagent [51] , [52] . In turn, these last two features enable the theoretical analysis of the labelling data of the homologous series of DP in order to quantify the number of defects for different g . As we shall discuss, the number of defects increases significantly for 1,000 PG6 thus suggesting the onset of SIS in the vicinity of g max . Importantly, the effects are evident only in the long 1,000 PG g but not in the short 45 PG g . This supports the SIS interpretation as defect accumulation due to imperfect reaction conversion should affect all DP irrespective of N . In contrast, SIS effects in the g range explored are envisioned only in long, locally cylindrical DP because of their lower g max . They are not expected in the 45 PG g series because of their higher g max arising since short DP adopts a dendrimer-like, near spherical, shape traceable to backbone end effects. Synthesis The divergent synthesis of a dendron proceeds from a f -functional root attached to a point-like core, to a linear polymer chain or to a surface (Fig. 2 and Supplementary Fig. S1 ). The roots are reacted with X -functional dendronization units (D units), having one reactive functionality and X −1 blocked, non-reactive, functional groups. In the next step, the blocked groups of the D units bound to the root are activated and their deblocked groups reacted with newly added D units. A g generation dendron is generated by g iterations of the deblocking reaction sequence. The generation g of the dendron thus specifies the maximal number of branching sites, junctions, along a strand joining the root to a terminal group. In the following, we focus on D units having the overall structure of a dendron junction or, equivalently, a g =1 dendron. In other words X is the functionality of the D unit, as well as the number of ‘arms’ emanating from a junction. In an ideal, structurally perfect g generation dendron each terminal junction bears X −1 blocked functionalities and every interior junction involves X bonds between chemically linked D units. Stated differently, the ideal structure contains no free functionalities that is, all functionalities are either blocked or covalently bound to another D unit. In a non-ideal dendron, some of the unblocked functionalities are not reacted and remain free and active ( Figs 1 and 2 ). Additionally, some may undergo side reactions rendering them inactive. 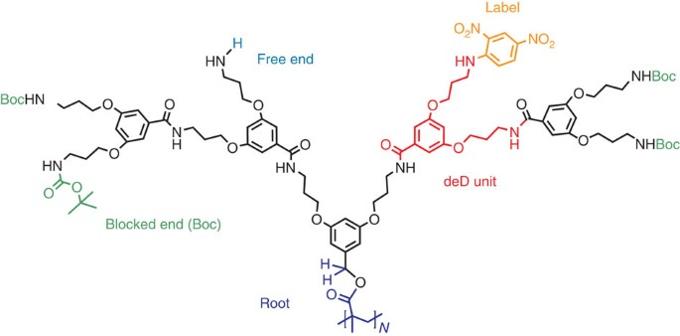Figure 1: Structural motifs of our dendrons. The chemical structure of theg=3,X=3,f=1 repeat unit ofNPG3 depicting the structural motifs invoked in the analysis: a root, blocked ends, a free end, a bound label and the deD unit forming an internal junction. This structure contains two defects, associated with strands containingg=2 junctions. It contains both a labelled and a free end, although in our discussion of theg≤gmaxrange we assume that all ends are quantitatively labelled and the two motifs may coexist only forg>gmax. The structures utilized for calculating the characteristic MM of the dendron are colouredM0=71.1 g mol−1(blue),=249.29 g mol−1(red),=101.12 g mol−1(green) and=167.1 g mol−1(orange). Note that the rootM0incorporates non-contiguous contributions so as to allow specifying the MM of theg=1 junction by a single. This definition differs from the customary convention. Figure 1: Structural motifs of our dendrons. The chemical structure of the g =3, X =3, f =1 repeat unit of N PG3 depicting the structural motifs invoked in the analysis: a root, blocked ends, a free end, a bound label and the deD unit forming an internal junction. This structure contains two defects, associated with strands containing g =2 junctions. It contains both a labelled and a free end, although in our discussion of the g ≤ g max range we assume that all ends are quantitatively labelled and the two motifs may coexist only for g > g max . The structures utilized for calculating the characteristic MM of the dendron are coloured M 0 =71.1 g mol −1 (blue), =249.29 g mol −1 (red), =101.12 g mol −1 (green) and =167.1 g mol −1 (orange). Note that the root M 0 incorporates non-contiguous contributions so as to allow specifying the MM of the g =1 junction by a single . This definition differs from the customary convention. 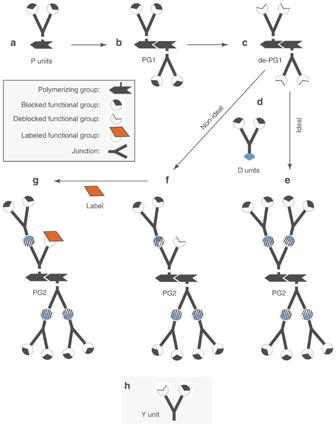Figure 2: Schematic view of the synthesis and labelling of DP. P units carrying each two blocked functionalities (a) are polymerized to form PG1. As P units are purified, the PG1 is structurally perfect. Conceptually it is useful to consider a polymer backbone withf-functional blocked repeat units that is then deblocked and reacted to form a PG1. (b) The resulting polymer is deblocked (c) and reacted with blocked D units (d) to yield PG2. In the ideal case (e) all deblocked functionalities are reacted. In reality, certain deblocked functionalities do not react and give rise to free ends (f). The amount of free ends is quantified by the absorbance of a labelling agent selectively binding them (g). Since the number of terminal groups in a highgideal DP is comparable to the number of inner D units, the typical MM of a branching unit corresponds to a Y unit (h). Full size image Figure 2: Schematic view of the synthesis and labelling of DP. P units carrying each two blocked functionalities ( a ) are polymerized to form PG1. As P units are purified, the PG1 is structurally perfect. Conceptually it is useful to consider a polymer backbone with f -functional blocked repeat units that is then deblocked and reacted to form a PG1. ( b ) The resulting polymer is deblocked ( c ) and reacted with blocked D units ( d ) to yield PG2. In the ideal case ( e ) all deblocked functionalities are reacted. In reality, certain deblocked functionalities do not react and give rise to free ends ( f ). The amount of free ends is quantified by the absorbance of a labelling agent selectively binding them ( g ). Since the number of terminal groups in a high g ideal DP is comparable to the number of inner D units, the typical MM of a branching unit corresponds to a Y unit ( h ). Full size image An iterative relationship between the numbers of junctions and of the free or blocked ends As the theoretical analysis is applicable to dendrimers as well as DP of different chemistries, we formulate it in general terms. Our theory considerations concern ‘elementary dendritic motifs’: a dendrimer, a repeat unit of a DP comprising of a root with the attached dendrons and the corresponding unit in a dendronized surface. We focus on the simplest case where there are no side reactions and the defects consist of free non-reacted functional groups, ‘free ends’. In this case, the structure of generation g dendritic motif is specified by the number of junctions n g , together with the number of blocked and free ends denoted respectively by and . The total number of ends, free or blocked, in generation g dendritic motif is = + . In turn, = f +( X −2) n g as the functionality of the root is f and each additional junction eliminates one functionality while contributing X −1 additional ones. The number of additional junctions generated with the g th synthesis step is denoted by Δ n g ≡ n g − n g −1 . In a generation g dendritic motif there are n g −1 ‘non terminal’, inner junctions. All Δ n g ‘new’ junctions are terminal junctions comprising of attached D units each with ( X −1) blocked functionalities. Accordingly, the number of blocked terminal functionalities in a dendritic motif of generation g is =( X −1)Δ n g . Combining =( X −1)( n g − n g −1 ) with the earlier relationships yields the key recursive equation relating n g , n g −1 and in a dendritic motif of a given X and f ( Fig. 3 ). It applies to the values characterizing individual dendritic motifs, as well as to ensemble averages denoted by ‹..›. Our key result is based on the utilization of Equation (1) to relate ‹ n g ›, ‹ n g −1 › and ‹ › of a homologous series of . In this case, it is possible to iteratively solve equation (1) and to obtain from labelling data providing partial information on ‹ ›, ..., , together with the initial values ‹ n 0 ›=‹ ›=0. Importantly, the complete set of ‹ n g › thus obtained fully specifies the corresponding ‹Δ n g ›, ‹ › and ‹ ›. 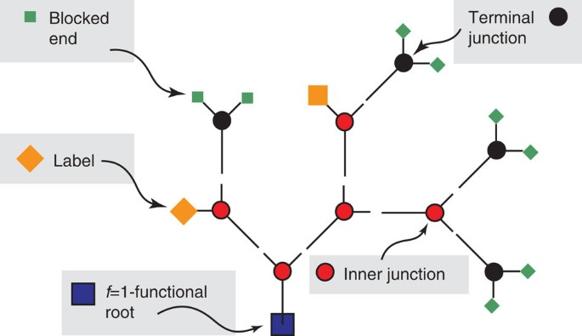Figure 3: Recursive relationships. A schematic view of a possibleg=4,X=3,f=1 DP dendron depicting=2 labelled ends,=8 blocked ends, Δn4=4 terminal junctions andn3=5 inner junctions. When=these quantities obey the following general relationships:n4=n3+Δn4,=(X−1)Δn4,=f+(X−2)n4andn4=(X−1)n3+f−. Figure 3: Recursive relationships. A schematic view of a possible g =4, X =3, f =1 DP dendron depicting =2 labelled ends, =8 blocked ends, Δ n 4 =4 terminal junctions and n 3 =5 inner junctions. When = these quantities obey the following general relationships: n 4 = n 3 +Δ n 4 , =( X −1)Δ n 4 , = f +( X −2) n 4 and n 4 =( X −1) n 3 + f − . Full size image Theoretical analysis of a labelling experiment To obtain ‹ n g › for the homologous series, we utilize labelling experiments where we measure two concentrations. The first is the molar concentration of labels bound to dendritic molecules of each generation, . For the case of efficient labelling reagent considered, we assume that all free ends are labelled and the number of labelled ends per dendritic motif is = . We note that this assumption is tenable only for g g max . For g > g max the free ends at the dendritic interior may be inaccessible to the labels thus leading to < . The onset of this effect depends on the size distribution of dendron voids, the size of the label and its interactions. The second measured quantity is the mass concentration of dendritic molecules w / V as specified by the weight of the dry labelled sample, w , and the solvent volume, V . In the following we convert the mass concentration to the molar concentration where M Y is a typical MM of a junction. M Y accounts for the contributions of both terminal junctions, bearing the two blocking groups, and internal junctions with no blocked groups ( Fig. 2 ): M Y = +( X −2) where is the MM of a chemically bound D unit within the ‘interior’ of the dendron and is the increment of MM of a blocking group bound to a deblocked D unit ( Fig. 1 ). and are both proportional to c g , the molar concentration of labelled dendritic motifs of generation g : = c g ‹ › and where ‹ › is the initially unknown average MM of a labelled dendritic motif of generation g . Their ratio, is thus independent of c g . U g is a rough estimate of ‹ ›/‹ n g › and it relates ‹ › to the yet to be specified ‹ ›. In turn, ‹ ›/ M Y is a linear function of ‹ n g › and ‹ n g −1 › with known coefficients A labelled , B labelled and C labelled (Methods and Fig. 1 ). This, together with equations (1) and (2) yields an iterative equation for ‹ n g ›, with the boundary condition ‹ n 0 ›=0, as specified by U 1 ,..., , the three coefficients determined by the chemical structure, as well as f and X (Methods, Fig. 1 ). For the particular DP investigated in this study, f =1 and X =3, hence A labelled ≈ 0.8117, B labelled ≈ 0.3766, and C labelled ≈ 0.6798 (Methods). Furthermore PG1 was obtained by polymerization of appropriate P units with f =1-functionality bound to a blocked D unit ( Fig. 2 ). Consequently, PG1 can be considered structurally perfect, corresponding to U 1 =0. Under these circumstances, the first two solutions of equation (3) are accordingly ‹ n 1 ›=1 and ‹ n 2 ›=[3− U 2 ( B labelled + C labelled )]/(1+ U 2 A labelled ). Higher g terms are obtained iteratively along the same lines. Analysis of the labelling measurements The results of the above analysis of the DP homologous series labelling data are depicted in plots of ‹ n g ›, ‹ › and ‹ › versus g for both the 1,000 PG g and 45 PG g series ( Figs 4 and 5 ). 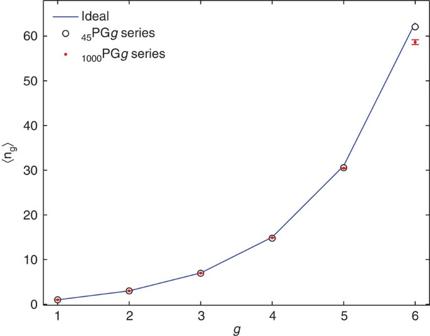Figure 4: Junctions per dendron for the members of the homologous series. The number of junctionsngversus the generationgfor both long1,000PGgand short45PGgseries as obtained from the labelling absorbance data upon using equation (3). In thegrange studied, the45PGgpoints are indistinguishable from the ideal values given by equation (4). In contrast, thengvalues of the1,000PG6 sample deviate from the ideal values. With the exception of1,000PG6 the error bars (s.d., Methods) are smaller than the symbols. The 45 PG1... 45 PG6 and 1,000 PG1... 1,000 PG5 are found to exhibit the behaviour of an ideal DP, Figure 4: Junctions per dendron for the members of the homologous series. The number of junctions n g versus the generation g for both long 1,000 PG g and short 45 PG g series as obtained from the labelling absorbance data upon using equation (3). In the g range studied, the 45 PG g points are indistinguishable from the ideal values given by equation (4). In contrast, the n g values of the 1,000 PG6 sample deviate from the ideal values. With the exception of 1,000 PG6 the error bars (s.d., Methods) are smaller than the symbols. 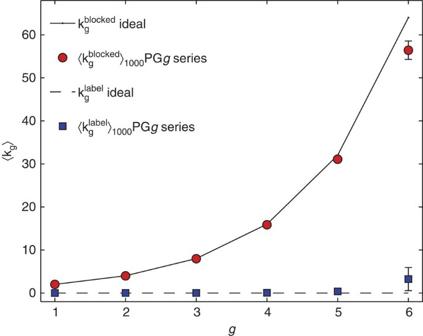Figure 5: Blocked and labelled ends per dendron. The number of blocked and labelled ends,andversus the generationgfor long1,000PGgas compared with the ideal values=f(X−1)gand=0 (depicted by lines). The1,000PG6 points deviate significantly from the ideal curves. In the 1≤g≤6 range, the45PGgvalues are indistinguishable from the ideal values and the corresponding points are not displayed. With the exception of1,000PG6 the error bars (s.d.) are smaller than the symbols. Full size image Figure 5: Blocked and labelled ends per dendron. The number of blocked and labelled ends, and versus the generation g for long 1,000 PG g as compared with the ideal values = f ( X −1) g and =0 (depicted by lines). The 1,000 PG6 points deviate significantly from the ideal curves. In the 1≤ g ≤6 range, the 45 PG g values are indistinguishable from the ideal values and the corresponding points are not displayed. With the exception of 1,000 PG6 the error bars (s.d.) are smaller than the symbols. Full size image equivalent to equation (3) when U g =0 for all g . In particular, ‹ ›/2 is indistinguishable from the number of terminal junctions in an ideal structure, = f ( X −1) g , and there are essentially no free ends, . In contrast, the 1,000 PG6 results deviate from this trend: ‹ n 6 ›< , ‹ ›< and ( Table 1 ). The onset of the deviations actually occurs at 1,000 PG5 as can be seen from the ‹ ›/‹ › versus g plot ( Fig. 6 ) that amplifies small deviations that are hard to discern in the ‹ › versus g plot. The upturn in the number of defects occurs below the estimated g max of this system, 6.1< g max <7.1 (ref. 50 ). However, the onset of packing effects is expected below g max because the densification of the system slows down transport with corresponding effect on the labelling kinetics. Importantly, the observed deviations occur only for the locally cylindrical 1,000 PG g series. There are no comparable effects for the 45 PG g homologous series, which exhibit ideal DP behaviour as specified by equation (4). This is an important observation supporting the interpretation of the data in terms of g max -related SIS effects. Two arguments are involved. The first concerns the N dependence of g max and the onset of SIS effects. For long locally cylindrical DP, the current estimate of g max of this chemistry vary in the 6.1< g max <7.1 range [50] and are thus consistent with onset of SIS at In contrast, short DP at high g exhibit dendrimer-like configurations because of backbone end effects. This suggests higher g max closer to 12.7< g max <14.1 estimated for dendrimers of similar chemistry [50] . Accordingly, g max effects are not expected for 45 PG1... 45 PG6. The second argument concerns the merits of an alternative explanation of the defect statistics in terms of imperfect conversion of the dendronization reactions. When excluding g max -dependent SIS effects, this second mechanism is expected to affect both 45 PG g and 1,000 PG g homologous series. The absence of such trend supports the interpretation in terms of SIS effects. Table 1 Defect characteristics deduced from labelling data of two homologous series. 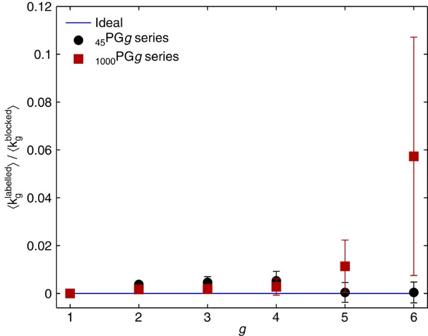Figure 6: Onset of branching defects. The ratio/amplifies the deviations from ideal behaviour at the price of larger error bars (s.d.). For short45PGg, the ratioas expected for an ideal DP and ideal dendrimer. In contrast long DPs deviate from ideal at1,000PG6 with an onset at1,000PG5. Full size table Figure 6: Onset of branching defects. The ratio / amplifies the deviations from ideal behaviour at the price of larger error bars (s.d.). For short 45 PG g , the ratio as expected for an ideal DP and ideal dendrimer. In contrast long DPs deviate from ideal at 1,000 PG6 with an onset at 1,000 PG5. Full size image Utilizing labelling technique we obtained evidence for the onset of SIS g max effects in long DP of g =6 g max close to 6.1< g max <7.1. This result is the first systematic confirmation of packing effects on the synthesis of dendritic molecules since their prediction in 1983. The attainment of g≈g max is also a first step towards the methodical exploration of g > g max dendritic molecules of interest as dense molecular objects with tunable size. Finally, the labelling technique, together with the theoretical framework reported, is a promising characterization technique for a significant family of dendritic molecules. As we shall discuss, it balances advantages, due to light instrumental and computational requirements, with shortcomings regarding its range of applicability. The labelling technique is applicable when four conditions are satisfied: (i) A homologous series of dendritic molecules is available. This is typically the case when utilizing divergent synthesis. (ii) The dominant defects are non-reacted, deblocked terminal groups. This is often the case for divergent synthesis using g =1 dendrons as D units. This condition is realized, for example, in Denkewalters dendritic peptides [17] , Newkomes arborols [18] and in Simaneks triazin-based dendrimers [53] . (iii) The defects can be efficiently interrogated by a labelling reagent. There is no universal label and the choice of the reagent should be customized to the synthetic chemistry used. When NH 2 groups are involved one may use the Sanger reagent [51] , [52] or Dansyl [54] , [55] , [56] . The Sanger reagent is less prone to aggregation and its smaller size is advantageous at high g . (iv) The labelling method can quantify all free ends for 1≤ g g max , that is, ‹ ›=‹ ›. For g > g max, it provides an efficient probe of exterior, accessible, free ends. However, the labels may encounter steric hindrance when binding defects situated within the dense dendritic interior that is,, ‹ ›<‹ ›. When these four requirements are met, the labelling method yields ‹ n g ›, ‹Δ n g ›, ‹ › and ‹ › for thus providing a complete characterization of the average structure. In particular, it specifies the average MM of the dendritic motif via equation (5) or its counterpart for the non-labelled moiety. MS when applicable, is free of these limitations [31] , [39] . However, it requires a dedicated facility and significant computational effort to deconvolute the spectra. In marked contrast, the labelling approach based on the Sanger method requires a ultraviolet spectrophotometer and minimal computational effort. With regard to MS and NMR, one should also note difficulties in characterizing high g dendritic molecules in general and DP in particular. These difficulties are even more pronounced for GPC. The interest in dendritic molecules is motivated in part by the vision of single-molecule colloidal particles of well-defined chemical structure. This direction is illustrated by 17,600 PG5, a single-molecule comparable in length and width to the potyvirus family and common cytoskeleton fibrils [48] , [57] . If one adheres to this point of view, it is important to establish g max because it signals the onset of SIS thus setting the upper boundary of synthetically attainable ideal dendritic molecules. However, the ‘post g max ’ regime may afford opportunities in spite of the unavoidable structural defects. Along the lines of the de Gennes–Hervet argument one may hypothesize that the structure of g > g max dendritic molecules is controlled by packing constraints resulting in dense molecules with well-defined dimensions. The investigation of this hypothesis again requires knowledge of g max , as well as efficient defect quantification methods for the g max range. Note that defects affect properties of dendritic molecules that depend on the number of end-groups, such as solubility. These observations confront a current lack of systematic observations of g max effects traceable to synthetic and characterization difficulties facing the exploration of the g max range. In this context, our work pioneers the synthesis of near g max DP and the quantitative exploration of the branching defects associated with SIS. It thus initiates the systematic investigation of the g ≳ g max regime. Synthesis of deblocked de - 1,000 PG5 Some of the starting material, denoted by 1,000 PG5, may have undergone charge-assisted, shear-induced main chain cleavage [58] , thus resulting in product of lower N . To a slowly- stirred, freeze-dried powder of 1,000 PG5 (0.20 g, 0.018 mmol repeat units) in a round bottom flask was dropwise added trifluoroacetic acid (TFA) (25 ml) and methanol (1 ml) at 0 °C. The reaction mixture soon turned homogeneous and was stirred at room temperature for 1 h. Then methanol (20 ml) was added and the mixture was evaporated in vacuo. This methanol addition and evaporation procedure was repeated twice, thereafter the residue was dissolved in water (15 ml) and carefully lyophilized to yield de - 1,000 PG5 as a powdery white solid (0.21 g, 100%). 1H NMR (500 MHz, DMF-d7): δ =0.90 (br, 18H, CH 3 ), 1.33 (br, 45H, CH 3 ), 2.01–2.19 (br, 326H, CH 2 ), 3.20–3.49 (br, 252H, CH 2 NH), 4.12 (br, 252H, CH 2 O), 6.42 (br, 75H, Ph), 7.08 (br, 142H, Ph), 8.41 (br, 30H, Ph, NH). Note: It is essential to avoid exposure of the de - 1,000 PG5 to shear forces because the chains can suffer a charge-assisted, shear-induced main chain cleavage [58] . Synthesis of blocked 1,000 PG6 To a dimethylformamide (DMF) solution (250 ml) of de - 1,000 PG5 (200 mg, 0.0174, mmol repeat unit) at −5 °C was added triethylamine (88 mg, 0.87 mmol) and N,N-dimethylaminopyridine (DMAP) (30 mg, 0.25 mmol). A solution of the D unit, the active ester dendron DG1 (3.15 g, 5.57 mmol) was added in six portions over 20 days. During the addition of each portion, the reaction mixture was cooled to −5 °C, then slowly warmed to room temperature and stirred for 3–4 days. After the addition of all the active ester dendron DG1, the reaction mixture was left stirring for another 10 days, then concentrated in vacuo. The residue was dissolved in 20 ml of dichloromethane (DCM) followed by column chromatography purification (eluent: DCM, Rf=0.1). This produced a beige gel, which was freeze-dried from 1,4-dioxane (40 ml) to yield 1,000 PG6 as a powdery, white solid (78 mg, 20%). 1H NMR (500 MHz, DMF-d7): δ =0.91 (br, 45H, CH 3 ),1.36 (br, 576H, CH 3 ), 1.89–2.02 (br, 273H, CH 2 ), 3.04 (br, 134H, CH 2 ), 3.18 (br, 153H, CH 2 ), 3.62 (br, 99H, CH 2 ), 4.08 (br, 252H, CH 2 ), 6.19 (br, 66H, CH), 6.58 (br, 79H, CH), 7.05 (br, 144H, CH), 8.16 (br, 45H, NH). Calcd for (C 1143 H 1654 N 126 O 318 ) N : C, 61.71; H, 7.49; N, 7.93. Found: C, 61.19; H, 7.20; N, 7.52. Synthesis of 45 PG1… 45 PG6 45 PG1 was synthesized by a reversible addition-fragmentation chain transfer (RAFT) protocol according to the reported procedure [59] . Divergent synthesis of 45 PG2... 45 PG6: to a solution of deprotected polymer precursor de - 45 PG( g -1) in DMF was added 4-dimethylaminopyridine (DMAP, cat.) and triethylamine (TEA, 2 eq. per amine) at −5 °C. Dendron active ester DG1 (5 eq. per amine) was added in three portions over a total predetermined time (4–15 days). Each portion was added at −5 °C, followed by a stirring at room temperature for 1–5 days. After the addition of the last portion and stirring, the reaction mixture was concentrated in vacuo. The residue was dissolved in DCM and purified by column chromatography (silica gel, DCM eluent) to give a beige gel, which was lyophilized from 1,4-dioxane to yield the product 45 PG g as a white powder (71–88%). Normalized GPC elution curves of 45 PG1... 45 PG6 are provided in Supplementary Fig. S2 . Labelling the DP To a well-stirred solution of blocked DP (5.0 mg) in 1,1,2,2-tetrachloroethane (0.3 ml) was added 0.1 M NaHCO 3 solution (0.043 ml), and a solution of Sanger reagent (0.4 mg, 0.3 eq. per Boc) was added in 1,1,2,2-tetrachloroethane (0.04 ml). The reaction mixture was stirred at 65 °C for 3 h, and then cooled to room temperature. 1,1,2,2-tetrachloroethane (2 ml), water (2 ml) and citric acid (1 mg) were added to the mixture. The organic layer was separated, washed by water (1 ml) and brine (1 ml), and concentrated in vacuo. The residue was dissolved in tetrahydrofuran (1 ml) and precipitated into methanol/water (4:1). This procedure was repeated four times to yield the labelled polymer in the form of a yellow solid (3.5 mg, 70%). Ultraviolet absorbance measurements Measurements ( Fig. 7 ) were performed on a Perkin Elmer Lambda 20 and a Jasco V-670 ultraviolet–vis spectrometer using 1 mm or 2 mm quartz cells, respectively. The labelled 1,000 PG6 was dissolved homogeneously in 1,1,2,2-tetrachloroethylene. The extinction coefficient ε =1.64 × 10 4 l mol −1 cm −1 (ref. 52 ) was assumed for 2,4-dinitroaniline moieties. Their concentration was calculated using the Lambert–Beer law ( c labelled = A /ε l ), in which l =0.1 cm ( 1,000 PG g ) or l =0.2 cm ( 45 PG g ) denotes the interior width of the quartz cell and A the absorbance at wave length λ =384 nm ( Fig. 7 ). 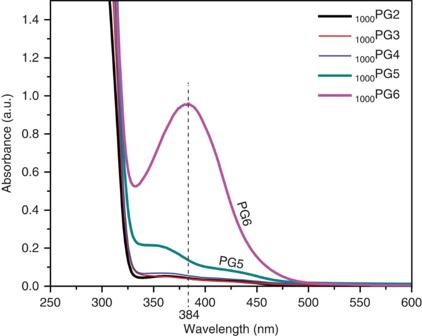Figure 7: Experimental labelling data. Plots of the ultraviolet absorbance (A) versus wave length for1,000PG2...1,000PG6.Ugis calculated fromAatλ=384 nm (dashed line), the location of the local maximum of the PG6 curve. a.u., arbitrary unit. Figure 7: Experimental labelling data. Plots of the ultraviolet absorbance ( A ) versus wave length for 1,000 PG2... 1,000 PG6. U g is calculated from A at λ =384 nm (dashed line), the location of the local maximum of the PG6 curve. a.u., arbitrary unit. Full size image Derivation of equation (3) The dimensionless coefficients A labelled , B labelled and C labelled occurring in are determined uniquely by the chemical structure All masses entering equation 6 had been introduced in Fig. 1 . Equation (5) with equation (6) follows from the mass accounting relationship = M 0 + n g + + upon substituting =( X −1)( n g − n g −1 ) and allowing for = + = f +( X −2) n g . Insertion of ‹ ›= U g [ A labelled ‹ n g ›+ B labelled ‹ n g −1 ›+ C labelled ] into equation (1) leads to equation (3). Error estimates The masses of the labelled polymer samples, w , and masses of the solution, w s , were measured up to a precision of δw =0.1 mg and δw s =10 mg, respectively, taking into account both instrumental and evaporation errors. The volumes of the polymer solutions are calculated from the measured masses, V = w s / ρ with ρ =(1.597±0.001)g cm −3 assuming the density of the dilute polymer solution is identical with that of the pure solvent ( Table 2 ). The molar concentrations of labels = A / ε l had been determined from the ultraviolet adsorbances A that come with a maximal relative error of 2% for the 45 PG g series (measured with Jasco V-670 (ref. 60 )), and 4% for the 1,000 PG g series (Perkin Elmer Lambda 20 (refs 48 , 15 )). The error of the denominator follows from δε≈ 100 (ref. 52 ) and δl≈ 1 micron. The relevant ratios Table 2 Summary of measured raw data and derived defect characteristics for the 45 PG g and 1,000 PG g series. Full size table furthermore involve our reference mass of a typical branching unit, M Y =(350.415±0.001) g mol −1 . The relative error δU g / U g thus follows immediately from the reported values in Table 2 and their above-mentioned errors by summing up the relative errors for all quantities on the rhs of equation 7. The calculation of ‹ n g › via the iterative relationship (equation 3 with f =1 and X =3) involves the dimensionless constants A labelled , B labelled and C labelled . As the chemical structure of the ideal dendron is known exactly, the relative error of these three coefficients is negligible. ‹ n 1 ›=1 being error free as discussed within the Results section. The error of ‹ n g › remains to be determined for given value and error of the preceding ‹ n g −1 › and the calculated U g ± δU g . Fortunately, the errors δU g occur in combinations of the form 1+ A labelled U g . Importantly, because δU g <<1 and because all coefficients A labelled , B labelled and C labelled are of order unity, the relative error δ ‹ n g › is mainly determined by ( X −1) δ ‹ n g −1 › alone, and does not grow exponentially. Furthermore, for g =4 or higher, when ‹ n g −1 ›>>1, the last bracket in the nominator of equation 8 becomes clearly irrelevant. If we denote the absolute error of ‹ n g › with δ ‹ n g › its relative error is with coefficients For example ( g =2): As ‹ n 1 ›=1, and this yields ≈ 1.2 × δU 1 for the numerical values of A labelled , B labelled and C labelled that are specified after equation 3. How to cite this article: Zhang, B. et al . Synthetic regimes due to packing constraints in dendritic molecules confirmed by labelling experiments. Nat. Commun. 4:1993 doi: 10.1038/ncomms2993 (2013).